Klf4 and Klf5 differentially inhibit mesoderm and endoderm differentiation in embryonic stem cells Krüppel-like factors (Klf) 4 and 5 are two closely related members of the Klf family, known to play key roles in cell cycle regulation, somatic cell reprogramming and pluripotency. Here we focus on the functional divergence between Klf4 and Klf5 in the inhibition of mouse embryonic stem (ES) cell differentiation. Using microarrays and chromatin immunoprecipitation coupled to ultra-high-throughput DNA sequencing, we show that Klf4 negatively regulates the expression of endodermal markers in the undifferentiated ES cells, including transcription factors involved in the commitment of pluripotent stem cells to endoderm differentiation. Knockdown of Klf4 enhances differentiation towards visceral and definitive endoderm. In contrast, Klf5 negatively regulates the expression of mesodermal markers, some of which control commitment to the mesoderm lineage, and knockdown of Klf5 specifically enhances differentiation towards mesoderm. We conclude that Klf4 and Klf5 differentially inhibit mesoderm and endoderm differentiation in murine ES cells. Klfs are evolutionarily conserved zinc-finger-containing transcription factors implicated in many biological processes, including proliferation, apoptosis, differentiation and development [1] . Klf4 and Klf5 are two closely related members of the Klf family that have a similar tissue distribution in embryos and adults. Yet Klf4 and Klf5 exert opposite effects on gene regulation [2] , [3] . They have been shown to antagonize each other in controlling expression of some target genes, despite sharing very similar, if not identical, cis -DNA sequences. A potential reason for this antagonistic effect is the physical competition of the two proteins in binding to a common cognate sequence [4] , [5] , [6] . Klf4 and Klf5 also exert contrasting effects on cellular proliferation. Klf4 is a growth arrest-associated gene involved in maintaining the integrity of the cell cycle [2] . It was shown to be necessary and sufficient for mediating the checkpoint function of p53 at both the G1/S and the G2/M transitions [7] . Klf4 is also a potential tumour suppressor in colorectal cancer [8] . In contrast to the growth inhibitory effect of Klf4, Klf5 exerts a growth promoting effect in cultured cells by activating the expression of the cell cycle regulators cyclin D1 and B1 as well as Cdk1 (ref. 2 ). Klfs received renewed attention after the demonstration that somatic cells could be reprogrammed into so-called induced pluripotent stem cells, using a cocktail of transcription factors that included KLF4 (ref. 9 ). A large body of evidence now indicates that expression of Klf4 and Klf5 genes is associated with pluripotency control. Both are highly expressed in mouse embryonic stem (ES) cells and their expression drops dramatically after induction of differentiation [10] , [11] . Expression of Klf4 and Klf5 is regulated by leukaemia inhibitory factor (LIF) via signal transduction and activator of transcription (STAT) 3 (ref. 10 ). Functional inactivation of either gene by RNA interference in ES cells induces spontaneous differentiation [10] , [12] , whereas overexpression reinforces self-renewal and delays differentiation induced by the formation of embryoid bodies (EBs) [12] , [13] . Klf5 −/− embryos fail to develop beyond the blastocyst stage in vivo and to produce ES cell lines in vitro [14] , a finding consistent with the Klf5 control of the pluripotency of epiblast, the embryonic tissue from which ES cells originate [15] . Klf4 −/− embryos develop to term [16] , suggesting that some compensatory mechanisms are able to rescue Klf4 function during early embryo development. How Klf4 and Klf5 regulate ES cell pluripotency is still not clear. They have been shown to regulate the expression of Nanog [17] , a pluripotency-associated gene involved in the inhibition of differentiation into primitive endoderm (PE) [18] , [19] , [20] , a finding consistent with the capacity of Klf4 and Klf5 to reinforce self-renewal when overexpressed [12] , [13] , [14] . We showed that Klf4 and Klf5 are both target genes of Nanog and STAT3 and that they can be equally activated by either factor [10] , a finding consistent with the capacity of Nanog to rescue endomesoderm differentiation induced by inactivation of the LIF/STAT3 pathway [18] , [19] . Studies based on chromatin immunoprecipitation (ChIP) coupled with a microarray assay or ultra-high-throughput DNA sequencing (ChIP-seq) revealed that Klf4 and Klf5 share many common targets. This further suggests the existence of a close functional relationship between these two factors [17] , [21] , [22] . Furthermore, they exhibit a high proportion of specific targets, which suggests functional divergence as well [23] . None of the reports examining the function of Klf factors in ES cells addressed directly the question of whether Klf4 and Klf5 play distinct roles in the control of pluripotency. Here we explored this issue by examining the phenotypes of ES cells in which the expression of Klf4 and Klf5 had been experimentally up- or downregulated. We show that knockdown of Klf4 upregulates the expression of endodermal markers and enhances the differentiation towards visceral and definitive endoderm. In contrast, knockdown of Klf5 upregulates the expression of mesodermal markers, and enhances the differentiation towards mesoderm. We conclude that Klf4 and Klf5 differentially inhibit mesoderm and endoderm differentiation in murine ES cells. Klf4 and Klf5 target genes in undifferentiated ES cells We started by analysing the changes in whole-genome expression profiles induced by Klf4 and Klf5 knockdown in undifferentiated ES cells. CGR8 ES cells were infected with five interfering lentiviral vectors: two vectors expressing two independent small hairpin RNA (shRNA) to Klf4 , two expressing two independent shRNA to Klf5 , and one expressing a control shRNA. All cells, hereafter called Klf4-KD1, Klf4-KD2, Klf5-KD1, Klf5-KD2 and control-KD, respectively, were subsequently cultured for 10 days at high density (≥5.10 4 cells per cm 2 )—to minimize spontaneous differentiation—in medium supplemented with G418 to kill the non-infected cells. Under such culture conditions, the resulting G418-resistant cell population showed twofold reductions in Klf4 and Klf5 transcript levels ( Fig. 1a ). However, they exhibited no sign of differentiation, as evidenced by the expression of pluripotency markers, Nanog , Oct4 ( pou5f1 ) and Rex1 ( Fig. 1a ), the percentage of SSEA-1 + cells ( Fig. 1b ), and the cell morphology ( Fig. 1c ). 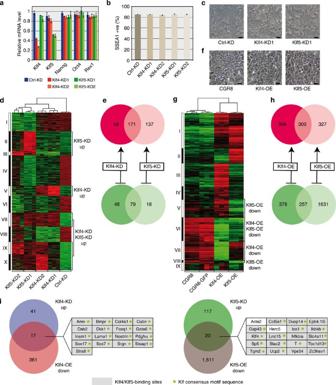Figure 1: Whole-transcriptome analysis of ESCs upon attenuation or reinforcement ofKlf4andKlf5expression. (a) Real-time PCR analysis ofKlf4,Klf5,Oct4,NanogandRex1expression in ES cells stably expressingKlf4,Klf5and control (GFP) shRNAs. Expression levels were normalized to control. (b) Histogram showing the percentage of SSEA-1+cells in the populations of ES cells expressingKlf4,Klf5,and control shRNAs. (c) Morphology of the ES cells expressingKlf4,Klf5and control shRNAs. Scale bar, 10 μm. (d) K-means clustering of differentially expressed probe sets (ANOVA, 5% false-discovery rate) in ES cells expressingKlf4,Klf5,and control shRNAs. Clusters II, III and V contain probe sets that were upregulated afterKlf4knockdown (cluster II and III) and downregulated after Klf5 knockdown (cluster V). Clusters VII, IX and X contain probe sets that were upregulated after bothKlf4andKlf5knockdown. Of note is that each group of probe sets resulted in more than one cluster. This finding results from differences in gene expression profiles after knockdown with two different shRNAs. (e) Venn diagrams of the genes up- and downregulated afterKlf4andKlf5knockdown in ES cells. (f) Morphology of the ES cells overexpressingKlf4andKlf5.Scale bar, 10 μm. (g) K-means clustering of differentially expressed probe sets (ANOVA) in ES cells overexpressingKlf4andKlf5and in control cells. (h) Venn diagrams of the genes up- and downregulated afterKlf4andKlf5overexpression in ES cells. (i) Venn diagrams illustrating the intersection between the lists of genes downregulated in Klf4-OE and Klf5-OE and the lists of genes upregulated in Klf4-KD and Klf5-KD, respectively. Genes displayed in a grey box were identified as target loci of Klf4 and Klf5 in the ChIP-seq experiment. Genes with a star display consensus Klf4/5 binding sites in their promoter sequence. (a,b) Mean and s.d. values were calculated from three biological replicates. Figure 1: Whole-transcriptome analysis of ESCs upon attenuation or reinforcement of Klf4 and Klf5 expression. ( a ) Real-time PCR analysis of Klf4 , Klf5 , Oct4 , Nanog and Rex1 expression in ES cells stably expressing Klf4 , Klf5 and control ( GFP ) shRNAs. Expression levels were normalized to control. ( b ) Histogram showing the percentage of SSEA-1 + cells in the populations of ES cells expressing Klf4 , Klf5, and control shRNAs. ( c ) Morphology of the ES cells expressing Klf4 , Klf5 and control shRNAs. Scale bar, 10 μm. ( d ) K-means clustering of differentially expressed probe sets (ANOVA, 5% false-discovery rate) in ES cells expressing Klf4 , Klf5, and control shRNAs. Clusters II, III and V contain probe sets that were upregulated after Klf4 knockdown (cluster II and III) and downregulated after Klf5 knockdown (cluster V). Clusters VII, IX and X contain probe sets that were upregulated after both Klf4 and Klf5 knockdown. Of note is that each group of probe sets resulted in more than one cluster. This finding results from differences in gene expression profiles after knockdown with two different shRNAs. ( e ) Venn diagrams of the genes up- and downregulated after Klf4 and Klf5 knockdown in ES cells. ( f ) Morphology of the ES cells overexpressing Klf4 and Klf5. Scale bar, 10 μm. ( g ) K-means clustering of differentially expressed probe sets (ANOVA) in ES cells overexpressing Klf4 and Klf5 and in control cells. ( h ) Venn diagrams of the genes up- and downregulated after Klf4 and Klf5 overexpression in ES cells. ( i ) Venn diagrams illustrating the intersection between the lists of genes downregulated in Klf4-OE and Klf5-OE and the lists of genes upregulated in Klf4-KD and Klf5-KD, respectively. Genes displayed in a grey box were identified as target loci of Klf4 and Klf5 in the ChIP-seq experiment. Genes with a star display consensus Klf4/5 binding sites in their promoter sequence. ( a , b ) Mean and s.d. values were calculated from three biological replicates. Full size image The transcriptomes of Klf4-KD1, Klf4-KD2, Klf5-KD1 and Klf5-KD2 were compared with that of control cells, using Mouse Genome 430 2.0 arrays. K-means clustering of probe sets for transcripts differentially expressed between the five ES cell populations (5% false-discovery rate) resulted in 10 clusters corresponding to genes up- or downregulated under one or several conditions ( Fig. 1d ), a finding consistent with previous reports showing that Klf4 and Klf5 can function as both a transcriptional activator and repressor [3] , [24] . After elimination of unidentified probe sets, and using filtering of 1.5-fold change in expression (analysis of variance (ANOVA), P <0.05), 145 genes were found to be downregulated and 366 upregulated after Klf4 or Klf5 knockdown ( Fig. 1e ). We focused all subsequent studies on the upregulated genes. Fifty-eight genes were upregulated after Klf4 knockdown. The highest fold change was observed with the endodermal markers Dab2 (7.5-fold), Foxa2 (5.2-fold), Sox17 (4.2-fold), Gata6 (4-fold), Gata4 (2.1-fold), Amn (2.1-fold) and Sox7 (1.9-fold). Using the same criteria for inclusion, 137 genes were found upregulated after Klf5 knockdown. The highest fold change was observed with the mesendodermal/mesodermal marker T (3.6-fold). In a second step, we evaluated the global changes in gene expression profiles induced by overexpressing Klf4 and Klf5. To this end, CGR8 ES cells were infected with lentiviral vectors expressing mouse Klf4 and Klf5 (designated Klf4-OE and Klf5-OE) at a multiplicity of infection of 20, which resulted in ~80% of the cell population expressing the transgenes. The OE cells exhibited an undifferentiated morphology ( Fig. 1f ). Parental ES cells and ES cells infected with a green fluorescent protein lentiviral vector were used as controls. Whole-transcriptome analysis was performed on these cells, and K-means clustering of probe sets for transcripts differentially expressed between the four ES cell populations resulted in six clusters corresponding to genes up- or downregulated in Klf4-OE, Klf5-OE or both ( Fig. 1g ). We identified 378 genes downregulated exclusively in Klf4-OE, and 1,631 genes downregulated exclusively in Klf5-OE, compared with the control cells (filtering of 1.5-fold change in expression (ANOVA, P <0.05)) ( Fig. 1h ). We next intersected the list of 2,009 genes downregulated in Klf4-OE and Klf5-OE with the list of the 511 genes upregulated in Klf4-KD and Klf5-KD, respectively. Of these, 37 genes were common to both groups and were accordingly considered the most likely specific responders ( Fig. 1i ). We identified 17 genes whose expression was upregulated in Klf4-KD cells and downregulated in Klf4-OE cells ( Amnionless , Bmpr , Col4a1 , Cubn , Dab2 , Dkk1 , Foxq1 , Gata6 , Insm1 , Lama1 , Nostrin , Pdgfrα , Sox17 , Sox7 , Srgn , Steap1 and Stra8 ). Sox7 , Sox17 , Dab2 , Amn and Gata6 , are known to be involved in the early commitment of embryonal carcinoma cells, ES cells, and primitive ectoderm of the early post-implantation embryo, to primitive and/or definitive endoderm [25] , [26] , [27] , [28] , [29] , [30] , [31] . Lama1 , encoding laminin alpha1, is highly expressed in endodermal cells [31] . We also identified 20 genes whose expression is upregulated in Klf5-KD cells and downregulated in Klf5-OE cells ( Acta2 , Col5a1 , Dusp14 , Epb4.1l5 , Gap43 , Herc5 , Ica1 , Ikbkb , Klf4 , Lrrc15 , Nfkbia , Slc4a11 , Sp5 , Stac2 , T , Tbc1d13, Tgm2, Ucp2 , Vps54 and Zc3hav1 ). Acta2 is an early marker for smooth muscle cells. Col5a1 is expressed in the connective tissues. T is first expressed in the primitive streak, the mesendoderm, and the mesoderm during gastrulation [32] . In the last step, to identify the genomic binding site distribution of Klf4 and Klf5, we performed ChIP-seq assays in ES cells using antibodies against endogenous Klf4 and Klf5. A de novo motif analysis on all genomic loci bound by Klf4 and Klf5 identified a similar binding sequence for both factors that is GC-rich and has a CACCC consensus core DNA-binding sequence, which is in agreement with previous reports [33] ( Supplementary Fig. 1a ). A comparison of Klf4 and Klf5 binding sites showed an overlap between the two factors with 63% of all Klf4 peaks and 79% of all Klf5 peaks shared with Klf5 and Klf4, respectively ( Supplementary Fig. 1b ). The peak distribution showed a similar pattern for both factors with enrichment at intergenic, intronic and promoter regions as expected ( Supplementary Fig. 1c ). We then intersected our list of binding sites with the 37 up- or downregulated genes, candidates for direct regulation, and found evidence that 35 of them were bound by Klf4 and Klf5 ( Fig. 1i ). Collectively, these results indicate that Klf4 and Klf5 regulate the expression of genes associated with mesoderm and endoderm lineages in ES cells. Klf4 and Klf5 regulate endoderm and mesoderm lineage markers The microarray data led us to hypothesize that Klf4 and Klf5 could preferentially regulate the expression of endoderm and mesoderm lineage markers, respectively. To explore this issue further, we examined the mRNA level of a subset of ectoderm, mesoderm and endoderm early markers in the Klf4-KD, Klf5-KD and control-KD cells. To this aim, CGR8 ES cells were infected with the interfering lentiviral vectors aforementioned; two vectors expressing two independent shRNA to Klf4 , two expressing two independent shRNA to Klf5 and one expressing a control shRNA. Five clones were isolated, one for each shRNA to Klf4 and Klf5, and one for control shRNA. All four Klf4-KD and Klf5-KD clones showed a strong reduction in Klf4 and Klf5 protein levels, respectively ( Fig. 2a ). We observed that most of the endoderm markers studied ( Amn , Emp2 (epithelial membrane protein 2), Dab2 , Foxa2 , Fxyd3 , Hnf4α , Gata4 , Gata6 , Sox17 , Sox7 ) were significantly upregulated in Klf4-KD cells compared with those in both control and Klf5-KD cells ( Fig. 2b , note log scale; Fig. 2c , note linear scale). In contrast, the mesoderm markers ( Bmp2 , Eomes , Flk1 , Hand1 , Mixl1 , Msx2 and T ) were significantly upregulated in Klf5-KD cells compared with those in both control and Klf4-KD cells. Ectoderm markers showed no significant variation among the three cell types. 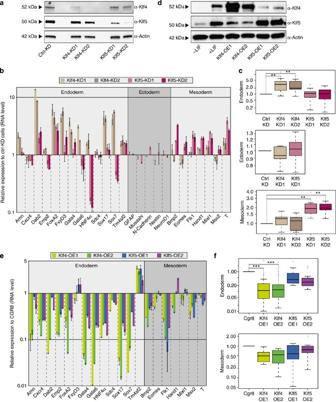Figure 2: Genes activated during the early steps of mesodermal and endodermal lineage commitment are differentially regulated byKlf4andKlf5in ESCs. (a) Western blot analysis of Klf4 and Klf5 expression in Klf4-KD1, Klf4-KD2, Klf5-KD1, Klf5-KD2 and control-KD clones. (b) Quantitative real-time PCR analysis of early ectodermal, mesodermal and endodermal markers in Klf4-KD, Klf5-KD and control ES cells. The histogram shows the mRNA level of the indicated genes in the four cell lines after normalization to control cells (note log scale). (c) Box plot representation of the mRNA level of endodermal, ectodermal and mesodermal markers shown in (b) (note linear scale). **P<0.01 using Kruskal–Wallis one way ANOVA. (d) Western blot analysis of Klf4 and Klf5 expression in Klf4-OE and Klf5-OE cells. +LIF indicates control cells. −LIF indicates control ES cells after withdrawal of LIF for 24 h. (e) Quantitative real-time PCR analysis of early mesodermal and endodermal markers in Klf4-OE, Klf5-OE and control cells. The histogram shows the mRNA level of the indicated genes in the four cell lines after normalization to control cells (note log scale). (f) Box plot representation of the mRNA level of endodermal and mesodermal markers, shown in (e) (note linear scale). ***P<0.001 using Kruskal–Wallis one way ANOVA. (b,e) Mean and s.d. values were calculated from three biological replicates. Figure 2: Genes activated during the early steps of mesodermal and endodermal lineage commitment are differentially regulated by Klf4 and Klf5 in ESCs. ( a ) Western blot analysis of Klf4 and Klf5 expression in Klf4-KD1, Klf4-KD2, Klf5-KD1, Klf5-KD2 and control-KD clones. ( b ) Quantitative real-time PCR analysis of early ectodermal, mesodermal and endodermal markers in Klf4-KD, Klf5-KD and control ES cells. The histogram shows the mRNA level of the indicated genes in the four cell lines after normalization to control cells (note log scale). ( c ) Box plot representation of the mRNA level of endodermal, ectodermal and mesodermal markers shown in ( b ) (note linear scale). ** P <0.01 using Kruskal–Wallis one way ANOVA. ( d ) Western blot analysis of Klf4 and Klf5 expression in Klf4-OE and Klf5-OE cells. +LIF indicates control cells. −LIF indicates control ES cells after withdrawal of LIF for 24 h. ( e ) Quantitative real-time PCR analysis of early mesodermal and endodermal markers in Klf4-OE, Klf5-OE and control cells. The histogram shows the mRNA level of the indicated genes in the four cell lines after normalization to control cells (note log scale). ( f ) Box plot representation of the mRNA level of endodermal and mesodermal markers, shown in ( e ) (note linear scale). *** P <0.001 using Kruskal–Wallis one way ANOVA. ( b , e ) Mean and s.d. values were calculated from three biological replicates. Full size image We performed a similar study with the Klf4-OE and Klf5-OE cells. Western blot analysis showed a strong increase in Klf4 and Klf5 protein levels in Klf4-OE and Klf5-OE, respectively ( Fig. 2d ). We observed that most of the endoderm markers were significantly downregulated in the Klf4-OE cells—but not in Klf5-OE cells—compared with those in both control and Klf5-OE cells (Kruskal–Wallis one way ANOVA, P <0.001). Endoderm markers were not significantly downregulated in Klf5-OE cells ( Fig. 2e , note log scale; Fig. 2f , note linear scale). In contrast, some of the mesoderm markers studied were downregulated in both Klf4-OE and Klf5-OE cells. Endogenous Klf4 and Klf5 ChIP-sequencing data allowed the identification of binding sites for both factors near all the genes found to be regulated by knockdown or overexpression of Klf4 and Klf5, including pluripotency genes Nanog and Oct4 , endodermal genes Gata6 , Sox17 , Amn , Cxcr4 , Dab2 , Emp2 , Foxa2 , Fxyd3 , Gata4 , HFN4α , Sdc4 and Sox7 , and mesodermal genes Mixl1 , Eomes , T , Flk1 , Bmp2 , Hand1 and Msx2 , as shown by the genome plots ( Supplementary Fig. 2 ). To relate binding of Klf4 and Klf5 at these sites with regulatory regions, we intersected our motif coordinates with sites defined by the ENCODE consortium for Bruce4 embryonic stem cells (ESCs) [34] , and examined the active promoter mark H3K4me3, the active enhancer mark H3K27Ac and the repressed promoter mark H3K27me3. We found that while for Nanog and Oct4 , Klf4 and Klf5 peaks overlapped with the active marks only, for endodermal and mesodermal genes, the peaks overlapped with both the active mark H3K4me3 and the repressive mark H3K27me3. In addition to endogenous Klf4 and Klf5, we performed ChIP-sequencing experiments in the Klf4-OE and Klf5-OE cells. A de novo motif analysis identified similar binding motifs for Klf4/Klf4-OE and Klf5/Klf5-OE factors ( Supplementary Fig. 1a ). Moreover, overexpressed Klf factors harboured a binding pattern similar to that of the endogenous factors at the aforementioned pluripotency, endodermal and mesodermal genes ( Supplementary Fig. 2 ), suggesting the absence of non-specific binding of the overexpressed Klfs. Collectively, all of these results strongly suggest that Klf4 preferentially regulates the expression of genes associated with endoderm differentiation, whereas Klf5 preferentially regulates the expression of genes associated with mesoderm differentiation. Klf4 and Klf5 differentially regulate lineage commitment Our finding that the expression of some genes associated with mesoderm and endoderm lineages was differentially regulated in Klf4-KD, Klf4-OE, Klf5-KD and Klf5-OE cells prompted us to study the role of Klf4 and Klf5 in endodermal versus mesodermal differentiation in vitro . For this purpose, Klf4 and Klf5 expression was knocked down with two lentiviral shRNA constructs for each gene, in two reporter ES cell lines, T-GFP-ES, expressing the enhanced green fluorescent protein under the regulatory elements of the mesoderm-specific T gene [35] , and Sox17-DsRed-ES, which expresses the DsRed fluorescent protein under the regulatory elements of the endoderm-specific Sox17 gene [36] . The infected cells were cultured at clonal density for 7 days. With each one of the two reporter cell lines, four clones exhibiting strong interference and one control clone were selected for all subsequent studies ( Fig. 3a ). Expression of the pluripotency markers Oct4 , Nanog and Rex1 was examined first, and revealed no significant differences between Klf4-KD, Klf5-KD and control cells. Furthermore, all clones analysed displayed the morphology of undifferentiated cells ( Fig. 3b ). This observation is consistent with a previous report that knockdown of a single Klf gene is not detrimental to self-renewal in high-density cultures [17] . All clones were induced to differentiate in suspension culture (EBs) for 1–10 days. Knockdown of Klf4 in the Sox17-DsRed-ES cells strongly increased the number of DsRed + cells at all the analysed time points (lowest increase (1.5-fold) was observed on day 10; highest increase (13.2-fold) was observed on day 2; average increase: 5.3-fold) ( Fig. 3c ; Supplementary Fig. 3a ). In contrast, knockdown of Klf4 in the T-GFP-ES cells moderately increased the number of GFP + cells (twofold on day 7). In a mirror image, knockdown of Klf5 in T-GFP-ES cells dramatically increased the number of GFP + cells (lowest increase (1.5-fold) was observed on day 4; highest increase (167.8-fold) was observed on day 6; average increase: 23.8-fold), whereas knockdown of Klf5 in Sox17-DsRed-ES cells did not alter the yield of DsRed + cells ( Fig. 3c ; Supplementary Fig. 3b ). Together, these observations suggest that the knockdown of Klf4 expression enhances commitment towards endoderm, whereas knockdown of Klf5 expression strongly enhances commitment towards mesoderm. 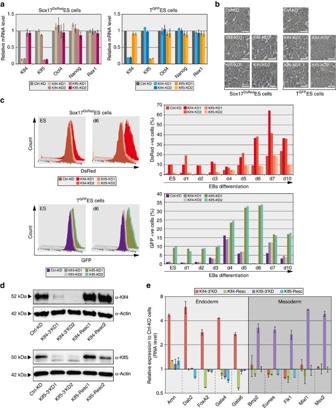Figure 3: Flow cytometry and quantitative real-time PCR analysis of endodermal and mesodermal differentiation after knockdown ofKlf4andKlf5expression. Sox17-DsRed and T-GFP reporter ES cell lines were infected withpLenti6/BLOCK-iT-PGKhygroR-lentiviral vectors expressing shKlf4-1, shKlf4-2, shKlf5-1 and shKlf5-2. After selection, hygromycin-resistant colonies were picked and analysed for the expression ofKlf4andKlf5by real-time PCR. Normalization was performed with β-actin. For each of the two reporter cell lines and each of the four vectors, two independent clones showing strong interference were selected. Clones expressing aKlf4/Klf5scrambled shRNA were engineered for control. Differentiation was induced by formation of EBs (day 1–day 10) in hanging drops. ES indicates undifferentiated ES cells. Data shown are from a representative experiment. (a) Quantitative real-time PCR analysis ofKlf4,Klf5,Oct4,NanogandRex1expression in the 5 T-GFP-ES and the 5 Sox17-DsRed-ES clones produced. Mean and s.d. values were calculated from three biological replicates. (b) Morphology of the cells in the 5 T-GFP-ES and the 5 Sox17-DsRed-ES clones. Scale bar, 10 μm. (c) Histogram representation of the percentage of DsRed+and GFP+cells during differentiation of Sox17-DsRed-ES and T-GFP-ES clones, respectively (results of a representative experiment). (d) Western blot analysis of Klf4 and Klf5 expression in Klf4-3′KD, Klf5-3′KD, Klf4-Resc, Klf5-Resc and control-KD cells. (e) Histogram showing the mRNA level of the indicated genes in Klf4-3′KD, Klf5-3′KD, Klf4-Resc and Klf5-Resc cell lines after normalization to control-KD cells (mean value measures each day from day 1 to day 7 of differentiation). Mean and s.d. values were calculated from two biological replicates. The results of the time-course experiment are shown inSupplementary Fig. 6. Figure 3: Flow cytometry and quantitative real-time PCR analysis of endodermal and mesodermal differentiation after knockdown of Klf4 and Klf5 expression. Sox17-DsRed and T-GFP reporter ES cell lines were infected with pLenti6/BLOCK-iT-PGKhygro R -lentiviral vectors expressing shKlf4-1, shKlf4-2, shKlf5-1 and shKlf5-2. After selection, hygromycin-resistant colonies were picked and analysed for the expression of Klf4 and Klf5 by real-time PCR. Normalization was performed with β-actin. For each of the two reporter cell lines and each of the four vectors, two independent clones showing strong interference were selected. Clones expressing a Klf4 / Klf5 scrambled shRNA were engineered for control. Differentiation was induced by formation of EBs (day 1–day 10) in hanging drops. ES indicates undifferentiated ES cells. Data shown are from a representative experiment. ( a ) Quantitative real-time PCR analysis of Klf4 , Klf5 , Oct4 , Nanog and Rex1 expression in the 5 T-GFP-ES and the 5 Sox17-DsRed-ES clones produced. Mean and s.d. values were calculated from three biological replicates. ( b ) Morphology of the cells in the 5 T-GFP-ES and the 5 Sox17-DsRed-ES clones. Scale bar, 10 μm. ( c ) Histogram representation of the percentage of DsRed + and GFP + cells during differentiation of Sox17-DsRed-ES and T-GFP-ES clones, respectively (results of a representative experiment). ( d ) Western blot analysis of Klf4 and Klf5 expression in Klf4-3′KD, Klf5-3′KD, Klf4-Resc, Klf5-Resc and control-KD cells. ( e ) Histogram showing the mRNA level of the indicated genes in Klf4-3′KD, Klf5-3′KD, Klf4-Resc and Klf5-Resc cell lines after normalization to control-KD cells (mean value measures each day from day 1 to day 7 of differentiation). Mean and s.d. values were calculated from two biological replicates. The results of the time-course experiment are shown in Supplementary Fig. 6 . Full size image The observed bias towards endoderm and mesoderm differentiation after knockdown of Klf4 and Klf5 , respectively, was confirmed by quantitative real-time PCR analysis of endoderm and mesoderm lineage markers in differentiating Sox17-DsRed cells ( Supplementary Fig. 4 ). The first group of factors marks differentiation into visceral and definitive endoderm [27] . They include Gata4 , Gata6 , Sox7 , Sox17 , Dab2 (Disabled-2), Foxa2 , Fxyd3 (FXYD protein 3), Cxcr4 , Sdc4 , Amn , Tm4sf2 and Emp2 , which all increased in Klf4-KD cells but not, or at a much reduced level, in Klf5-KD cells. The second group of genes marks commitment towards the mesendodermal lineage and/or differentiation into mesoderm. They include T , Mixl1 , Eomes , Hand1 , Msx2 , Bmp2 and Flk1 , which all increased in Klf5-KD cells, but not in Klf4-KD cells, relative to control. Compared with control cells, the third group includes genes that mark differentiation into neurectoderm ( Nestin, Musashi , N-cadherin , GFAP and NeuroD1 ), and which remained unchanged in Klf4-KD and Klf5-KD cells. The results of time-course experiments performed between day 0 and day 10 of EB differentiation are given in Supplementary Fig. 5 . Within a group of markers, differences are observed according to whether they are upregulated at all the analysed time points, or activated only at some time points. Differences are particularly striking within the group of endoderm markers, where some ( Gata4 , Gata6 , Sox17 , Amn , Dab2 ) were induced at all the analysed time points in Klf4-KD cells, whereas Foxa2 , Cxcr4 , Tm4sf2 , Sdc4 and Emp2 were induced only at late time points. Such differences in the pattern of marker expression in Klf4-KD cells suggests that some gene markers are upregulated as a direct consequence of Klf4 knockdown in early differentiating cells, whereas other markers are upregulated late possibly because they are secondary changes. Finally, we examined whether re-expressing shRNA-resistant Klf4 and Klf5 rescued the phenotype of Klf4-KD and Klf5-KD cells, respectively. To this goal, CGR8 ESCs were infected with four interfering lentiviral vectors expressing (i) two different shRNAs to the 3′untranslated region of Klf4 mRNA (shKlf4 3′UTR ), and (ii) two different shRNAs to the 3′untranslated region of Klf5 mRNA (shKlf5 3′UTR ). With each of the four interfering vectors, one clone exhibiting strong interference was selected. Each one of these four clones (designated Klf4-3′KD1, shKlf4-3′KD2, Klf5-3′KD1 and Klf5-3′KD2) was then infected with the above described lentiviral vectors expressing mouse Klf4 and Klf5. The expression level of Klf4 and Klf5 in the rescued lines was measured by western blot. Two clones, designated Klf4-Resc1 and Klf5-Resc1, showing an expression level of the Klf4 and Klf5 transgenes close to that of the wild-type ESCs, were selected for functional analysis ( Fig. 3d ). All clones were induced to differentiate in EBs for 1–7 days. For clarity, the mean value of the fold changes measured each day from day 1 to day 7 of differentiation is shown for each marker analysed ( Fig. 3e ). The results of the time-course experiment are shown in Supplementary Fig. 6 ). The five endodermal markers analysed ( Amn , Dab2 , Foxa2 , Gata4 and Gata6 ) showed increased expression in the Klf4-3′KD clone in accord with the results obtained with Klf4-KD cells. Their expression level was dramatically reduced in the Klf4-Resc1 cells. Similarly, the five mesodermal markers analysed ( Bmp2 , Eomes , Flk1 , Mixl1 and Msx2 ) showed increased expression in the Klf5-3′KD clone in accord with the results obtained with Klf5-KD cells. Their expression level was dramatically reduced in the Klf5-Resc1 cells. These results collectively indicate that knockdown of Klf4 expression results in increased differentiation towards endoderm, whereas knockdown of Klf5 expression enhances differentiation into the mesoderm lineage. Klf4 regulates commitment to endoderm Sox 17 , which we showed is regulated by Klf4, is expressed in extraembryonic visceral and definitive endoderm [37] , raising the question of whether Klf4 knockdown can interfere with the commitment of pluripotent ES cells into both types of endoderm. To answer this question, we made use of the ES-Gsc gfp Sox17 huCD25 reporter cell line, which bears the gfp and human CD25 marker genes in the goosecoid ( Gsc ) and Sox17 loci, respectively. Differential expression of these two markers distinguishes visceral endoderm (Gsc − Sox17 + ) from definitive endoderm (Gsc + Sox17 + ). The rare Gsc + Sox17 − cell population represents mesendoderm, which has been described in ESC culture [27] . We generated ES-Gsc gfp Sox17 huCD25 subclones, in which the expression of Klf4 and Klf5 was knocked down. Compared with control, the average expression level of Oct4 , Nanog and Rex1 was reduced by ~20% in the resulting ES-Gsc gfp Sox17 huCD25 -Klf4-KD and ES-Gsc gfp Sox17 huCD25 -Klf5-KD clones ( Fig. 4a ). However, no sign of differentiation could be observed ( Fig. 4b ). We next examined the capacity of these clones to differentiate into mesendoderm cells, and visceral and definitive endoderm lineages, in three differentiation protocols. In the first protocol, ES-Gsc gfp Sox17 huCD25 -Klf4-KD and ES-Gsc gfp Sox17 huCD25 -Klf5-KD clones were induced to differentiate by formation of EBs. Compared with control cells, ES-Gsc gfp Sox17 huCD25 -Klf4-KD clones exhibited an increased number of GFP − CD25 + cells (visceral endoderm), GFP + CD25 − cells (mesendoderm cells) and GFP + CD25 + cells (definitive endoderm) ( Fig. 4c,d ; Supplementary Fig. 7a . In contrast, ES-Gsc gfp Sox17 huCD25 -Klf5-KD clones exhibited no significant changes in the yield of visceral and definitive endoderm. These results are in agreement with, and extend, our previous findings that only Klf4 inhibits differentiation into endoderm lineages. In the second protocol, the cells were plated at a density of 10 4 cells per cm −2 in LIF-deprived serum-free medium to direct differentiation into visceral endoderm, as previously described [27] . ES-Gsc gfp Sox17 huCD25 -Klf4-KD cells exhibited an increased capacity to form visceral endoderm, further evidenced by the increased expression of the visceral endoderm-specific markers Amn and Pthr1 (ref. 27 ). Cxcr4 and Tm4sf2 , two markers of definitive endoderm, were not expressed under those culture conditions ( Fig. 4e,f ; Supplementary Fig. 7b ). In the third protocol, ES-Gsc gfp Sox17 huCD25 -Klf4-KD and ES-Gsc gfp Sox17 huCD25 -Klf5-KD clones were induced to differentiate in LIF-deprived serum-free medium supplemented with activin to direct differentiation into definitive endoderm [27] . Both ES-Gsc gfp Sox17 huCD25 -Klf4-KD clones showed a dramatically increased propensity to differentiate into definitive endoderm, further evidenced by the increased expression of the definitive endoderm-specific markers, Cxcr4 and Tm4sf2 [27] ( Fig. 4g,h ; Supplementary Fig. 7c ). In contrast, the ES-Gsc gfp Sox17 huCD25 -Klf5-KD clones showed no significant changes in the yield of visceral endoderm, and definitive endoderm. Of note, higher concentration of activin was tested to improve definitive endoderm differentiation in control, but resulted in massive cell death. These data are thus entirely consistent with those previously obtained after differentiation in suspension culture, and indicate that only the knockdown of Klf4 enhanced differentiation into both visceral and definitive endoderm. 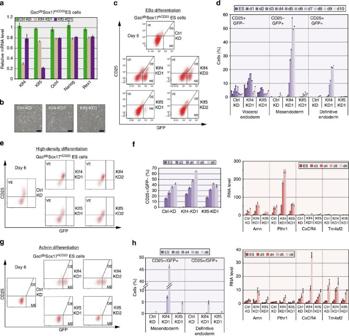Figure 4: Knockdown ofKlf4increases the yield of visceral and definitive endoderm. (a) Histogram representation of the relative mRNA levels forKlf4,Klf5,Oct4,NanogandRex1in ES-GscgfpSox17huCD25-Klf4-KD, ES-GscgfpSox17huCD25-Klf5-KD and control clones. Mean and s.d. were calculated from three technical replicates from on representative experiment. (b) Morphology of the ES-GscgfpSox17huCD25-Klf4-KD, ES-GscgfpSox17huCD25-Klf5-KD and control clones. Scale bar, 10 μm. (c,d) Differentiation induced by suspension culture (EB). (c) FACS profiles of ES-GscgfpSox17huCD25-Klf4-KD1, ES-GscgfpSox17huCD25-Klf4-KD2, ES-GscgfpSox17huCD25-Klf5-KD1, ES-GscgfpSox17huCD25-Klf5-KD2 and control cells, after immunostaining for CD25 expression, and showing increased differentiation to visceral endoderm (CD25+GFP−), mesendoderm (CD25−GFP+) and definitive endoderm (CD25+GFP+) from the ES-GscgfpSox17huCD25-Klf4-KD cells. (d) Histogram representation of the percentages of CD25+GFP−(visceral endoderm), CD25−GFP+(mesendoderm) and CD25+GFP+(definitive endoderm) cells during differentiation; d1 to d10 indicate days of differentiation. (e,f) Differentiation induced by high-density culture and LIF deprivation. (e) FACS profiles of ES-GscgfpSox17huCD25-Klf4-KD1, ES-GscgfpSox17huCD25-Klf4-KD2, ES-GscgfpSox17huCD25-Klf5-KD1, ES-GscgfpSox17huCD25-Klf5-KD2 and control cells, after immunostaining for CD25 expression, and showing increased differentiation to visceral endoderm (CD25+GFP−) from the ES-GscgfpSox17huCD25-Klf4-KD cells. (f) Left panel: histogram representation of the percentages of CD25+GFP−cells (visceral endoderm) during differentiation; d3 to d6 indicate days of differentiation. Right panel: histogram representation of the mRNA level ofAmn, andPthr1(visceral endoderm) andCxcr4andTm4sf2(definitive endoderm) measured by quantitative real-time PCR in ES-GscgfpSox17huCD25-Klf4-KD, ES-GscgfpSox17huCD25-Klf5-KD and control cells, during differentiation. (g,h) Differentiation induced by activin. (g) FACS profiles of FACS profiles of ES-GscgfpSox17huCD25-Klf4-KD1, ES-GscgfpSox17huCD25-Klf4-KD2, ES-GscgfpSox17huCD25-Klf5-KD1, ES-GscgfpSox17huCD25-Klf5-KD2, and control cells, after immunostaining for CD25 expression, and showing increased differentiation to mesendoderm (CD25−GFP+) and to definitive endoderm (CD25+GFP+) from the ES-GscgfpSox17huCD25-Klf4-KD cells. (h) Left panel: histogram representation of the percentages of CD25–GFP+cells (mesendoderm) and CD25+GFP+cells (definitive endoderm during differentiation; d3 to d6 indicate days of differentiation. Right panel: histogram representation of the mRNA level ofAmn, andPthr1(visceral endoderm) andCxcr4andTm4sf2(definitive endoderm) measured by quantitative real-time PCR in ES-GscgfpSox17huCD25-Klf4-KD, ES-GscgfpSox17huCD25-Klf5-KD and control cells, during differentiation. (d,f,h) Mean and s.d. values were calculated from three biological replicates. Figure 4: Knockdown of Klf4 increases the yield of visceral and definitive endoderm. ( a ) Histogram representation of the relative mRNA levels for Klf4 , Klf5 , Oct4 , Nanog and Rex1 in ES-Gsc gfp Sox17 huCD25 -Klf4-KD, ES-Gsc gfp Sox17 huCD25 -Klf5-KD and control clones. Mean and s.d. were calculated from three technical replicates from on representative experiment. ( b ) Morphology of the ES-Gsc gfp Sox17 huCD25 -Klf4-KD, ES-Gsc gfp Sox17 huCD25 -Klf5-KD and control clones. Scale bar, 10 μm. ( c,d ) Differentiation induced by suspension culture (EB). ( c ) FACS profiles of ES-Gsc gfp Sox17 huCD25 -Klf4-KD1, ES-Gsc gfp Sox17 huCD25 -Klf4-KD2, ES-Gsc gfp Sox17 huCD25 -Klf5-KD1, ES-Gsc gfp Sox17 huCD25 -Klf5-KD2 and control cells, after immunostaining for CD25 expression, and showing increased differentiation to visceral endoderm (CD25 + GFP − ), mesendoderm (CD25 − GFP + ) and definitive endoderm (CD25 + GFP + ) from the ES-Gsc gfp Sox17 huCD25 -Klf4-KD cells. ( d ) Histogram representation of the percentages of CD25 + GFP − (visceral endoderm), CD25 − GFP + (mesendoderm) and CD25 + GFP + (definitive endoderm) cells during differentiation; d1 to d10 indicate days of differentiation. ( e,f ) Differentiation induced by high-density culture and LIF deprivation. ( e ) FACS profiles of ES-Gsc gfp Sox17 huCD25 -Klf4-KD1, ES-Gsc gfp Sox17 huCD25 -Klf4-KD2, ES-Gsc gfp Sox17 huCD25 -Klf5-KD1, ES-Gsc gfp Sox17 huCD25 -Klf5-KD2 and control cells, after immunostaining for CD25 expression, and showing increased differentiation to visceral endoderm (CD25 + GFP − ) from the ES-Gsc gfp Sox17 huCD25 -Klf4-KD cells. ( f ) Left panel: histogram representation of the percentages of CD25 + GFP − cells (visceral endoderm) during differentiation; d3 to d6 indicate days of differentiation. Right panel: histogram representation of the mRNA level of Amn , and Pthr1 (visceral endoderm) and Cxcr4 and Tm4sf2 (definitive endoderm) measured by quantitative real-time PCR in ES-Gsc gfp Sox17 huCD25 -Klf4-KD, ES-Gsc gfp Sox17 huCD25 -Klf5-KD and control cells, during differentiation. ( g,h ) Differentiation induced by activin. ( g ) FACS profiles of FACS profiles of ES-Gsc gfp Sox17 huCD25 -Klf4-KD1, ES-Gsc gfp Sox17 huCD25 -Klf4-KD2, ES-Gsc gfp Sox17 huCD25 -Klf5-KD1, ES-Gsc gfp Sox17 huCD25 -Klf5-KD2, and control cells, after immunostaining for CD25 expression, and showing increased differentiation to mesendoderm (CD25 − GFP + ) and to definitive endoderm (CD25 + GFP + ) from the ES-Gsc gfp Sox17 huCD25 -Klf4-KD cells. ( h ) Left panel: histogram representation of the percentages of CD25 – GFP + cells (mesendoderm) and CD25 + GFP + cells (definitive endoderm during differentiation; d3 to d6 indicate days of differentiation. Right panel: histogram representation of the mRNA level of Amn , and Pthr1 (visceral endoderm) and Cxcr4 and Tm4sf2 (definitive endoderm) measured by quantitative real-time PCR in ES-Gsc gfp Sox17 huCD25 -Klf4-KD, ES-Gsc gfp Sox17 huCD25 -Klf5-KD and control cells, during differentiation. ( d , f , h ) Mean and s.d. values were calculated from three biological replicates. Full size image Klf5 regulates commitment to mesoderm We observed a strong increase in the yield of Gsc + Sox17 − cells (GFP + CD25 − cells, Fig. 4c ) after Klf4 knockdown, suggesting that Klf4 inhibits differentiation towards mesendoderm cells. This conclusion is reinforced by the observation that Klf4 knockdown results in a moderate increase in the percentage of GFP + cells in T GFP /Klf4-KD cells on day 7 of differentiation ( Fig. 3c ). This may be explained by the fact that expression of T begins in mesendoderm cells, before becoming restricted to the mesoderm lineage [38] . In contrast, Klf5 knockdown did not increase the yield of Gsc + Sox17 − mesendoderm cells ( Fig. 4c ), but it strongly increased the percentage of GFP + cells -Bra GFP /Klf5-KD cells ( Fig. 3c ). Klf5 knockdown also resulted in an elevation of expression of all mesoderm markers examined including Mixl1 , Flk1 , Hand1 and Msx2 . These observations led us to suggest that Klf5 interferes with the commitment of mesendoderm cells into mesoderm lineage. To address this question more directly, we examined the capacity of the Klf4-KD1, Klf4-KD2, Klf5-KD1 and Klf5-KD2 cell lines to differentiate into mesoderm using two differentiation protocols. In the first protocol, ESCs were induced to differentiate by formation of EBs. Compared with control cells, both Klf4-KD and Klf5-KD clones exhibited an increased number of Flk1 + E-Cadh − and PDGFRα + E-Cadh − cells (mesoderm). Most importantly, the observed increase appeared much stronger in the Klf5-KD clones. This result was observed at 6, 7 and 8 days of differentiation ( Fig. 5a,b ). The two Klf4-KD clones also showed strongly elevated numbers of endoderm cells (Flk1 − E-Cadh + and PDGFRα − E-Cadh + ). In contrast, the two Klf5-KD clones did not show such an elevation, in accordance with our previous results. In the second protocol, differentiation was performed in α modified Eagle’s medium to enhance mesoderm differentiation [39] . Under these conditions, only the Klf5-KD clones showed an increased number of Flk1 + E-Cadh − and PDGFRα + E-Cadh − mesodermal cells ( Fig. 5c,d ). 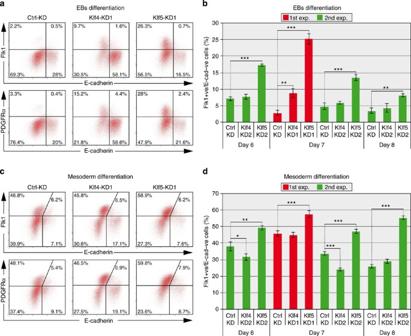Figure 5: Knockdown ofKlf5increases the yield of definitive mesoderm. (a) FACS profiles of Klf4-KD1, Klf4-KD2, Klf5-KD1, Klf5-KD2 and control cells (Ctrl-KD), after immunostaining for Flk1, PDGFRα and E-cadherin expression, and showing increased differentiation to mesoderm (Flk1+E-Cadh−and PDGFRα+E-Cadh−) in both Klf4-KD and Kf5-KD cells at day 7 of EB differentiation (differentiation in GMEM+10% fetal calf serum). (b) Histogram representation of the percentages of Flk1+E-Cadh−cells on days 6, 7 and 8 of EB differentiation in GMEM+10% fetal calf serum. **P<0.01; ***P<0.001, using Student’st-test. (c) FACS profiles of Klf4-KD1, Klf4-KD2, Klf5-KD1, Klf5-KD2 and control cells, after immunostaining for Flk1, PDGFRα and E-cadherin expression, and showing increased differentiation to mesoderm (Flk1+E-Cadh−and PDGFRα+E-Cadh−) in Klf5-KD cells on day 7 of EB differentiation (differentiation in α Modified Eagle’s Medium+5% fetal calf serum). (d) Histogram representation of the percentages of Flk1+E-Cadh−cells at days 6, 7 and 8 of EB differentiation in α Modified Eagle’s Medium+5% fetal calf serum. *P<0.05;**P<0.01; ***P<0.001 using Student’st-test. (b,d) Mean and s.d. values were calculated from three biological replicates. Figure 5: Knockdown of Klf5 increases the yield of definitive mesoderm. ( a ) FACS profiles of Klf4-KD1, Klf4-KD2, Klf5-KD1, Klf5-KD2 and control cells (Ctrl-KD), after immunostaining for Flk1, PDGFRα and E-cadherin expression, and showing increased differentiation to mesoderm (Flk1 + E-Cadh − and PDGFRα + E-Cadh − ) in both Klf4-KD and Kf5-KD cells at day 7 of EB differentiation (differentiation in GMEM+10% fetal calf serum). ( b ) Histogram representation of the percentages of Flk1 + E-Cadh − cells on days 6, 7 and 8 of EB differentiation in GMEM+10% fetal calf serum. ** P <0.01; *** P <0.001, using Student’s t -test. ( c ) FACS profiles of Klf4-KD1, Klf4-KD2, Klf5-KD1, Klf5-KD2 and control cells, after immunostaining for Flk1, PDGFRα and E-cadherin expression, and showing increased differentiation to mesoderm (Flk1 + E-Cadh − and PDGFRα + E-Cadh − ) in Klf5-KD cells on day 7 of EB differentiation (differentiation in α Modified Eagle’s Medium+5% fetal calf serum). ( d ) Histogram representation of the percentages of Flk1 + E-Cadh − cells at days 6, 7 and 8 of EB differentiation in α Modified Eagle’s Medium+5% fetal calf serum. * P <0.05;** P <0.01; *** P <0.001 using Student’s t -test. ( b , d ) Mean and s.d. values were calculated from three biological replicates. Full size image Collectively, these results indicate that knockdown of both Klf4 and Klf5 expression results in an enhancement of mesodermal differentiation. However, the effect of Klf5 knockdown is much stronger. Regulation of Gata6 and Mixl1 by Klf4 and Klf5 We observed that Gata6 mRNA level increased when Klf4 expression was attenuated, and decreased when Klf4 was overexpressed. Similarly, the Mixl1 mRNA level was found to increase when Klf5 expression was attenuated, and decreased when Klf5 was overexpressed. In addition, Klf4 and Klf5 were found to bind Gata6 and Mixl1 promoters. This observation was initially made by ChIP-seq ( Supplementary Fig. 2 ), and was confirmed by ChIP–PCR ( Fig. 6a ). To demonstrate that Klf4 and Klf5 regulate the expression of Gata6 and Mixl1 , respectively, we performed promoter studies. We observed that a luciferase-based Gata6 promoter reporter was strongly activated when co-transfected with a shKlf4 expression vector, in comparison with shKlf5 and control vectors ( Fig. 6b ). Similarly, the Gata6 promoter luciferase reporter was strongly activated in Klf4-KD1 cells in comparison with Klf5-KD1 and control cells ( Fig. 6c ). We also observed that a luciferase-based Mixl1 promoter was strongly activated when co-transfected with a shKlf5 expression vector, in comparison with shKlf4 and control vectors. Similarly, the Mixl1 promoter luciferase reporter was strongly activated in Klf5-KD1 cells, in comparison with Klf4-KD1 and control cells ( Fig. 6b,c ). Thus reducing the levels of Klf4 and Klf5 promotes Gata6 and Mixl1 promoter activity, respectively. Together, these results demonstrate that both Gata6 and Mixl1 are direct targets of Klf4 and Klf5. However, only Gata6 is regulated by Klf4, and only Mixl1 is regulated by Klf5. 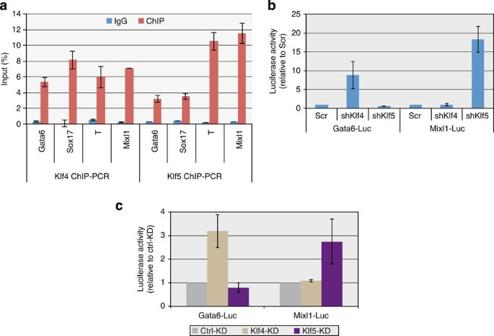Figure 6: Klf4 and Klf5 inhibit the promoters ofGata6andMixl1, respectively. (a) ChIP experiment using Klf4 and Klf5 antibodies in ESCs. Fold enrichments (relative to input DNA) were assessed at Klf4- and Klf5-binding sites in theGata6, Sox17, Mixl1andTpromoter regions. Mean and s.d. values were calculated from three technical replicates. (b) Transfection ofGata6andMixl1promoter luciferase reporters (pGL4-Gata6ProandpGL4-Mixl1Pro) with shKlf4, shKlf5 and control shRNA in ES cells. (c) Transfection ofpGL4-Gata6ProandpGL4-Mixl1Proin Klf4-KD1, Klf4-KD2 and control ES cells. (b,c) Histogram representation of luciferase activity after normalization toRenillaluciferase activity and to firefly luciferase activity measured with thepGL4.10 Luc2reporter plasmid (control). (b,c) Mean and s.d. values were calculated from three biological replicates. Figure 6: Klf4 and Klf5 inhibit the promoters of Gata6 and Mixl1 , respectively. ( a ) ChIP experiment using Klf4 and Klf5 antibodies in ESCs. Fold enrichments (relative to input DNA) were assessed at Klf4- and Klf5-binding sites in the Gata6, Sox17, Mixl1 and T promoter regions. Mean and s.d. values were calculated from three technical replicates. ( b ) Transfection of Gata6 and Mixl1 promoter luciferase reporters ( pGL4-Gata6Pro and pGL4-Mixl1Pro ) with shKlf4, shKlf5 and control shRNA in ES cells. ( c ) Transfection of pGL4-Gata6Pro and pGL4-Mixl1Pro in Klf4-KD1, Klf4-KD2 and control ES cells. ( b , c ) Histogram representation of luciferase activity after normalization to Renilla luciferase activity and to firefly luciferase activity measured with the pGL4.10 Luc2 reporter plasmid (control). ( b , c ) Mean and s.d. values were calculated from three biological replicates. Full size image Klf4 and Klf5 regulate lineage choice in teratomas We next investigated whether Klf4 and Klf5 knockdown exerts a similar bias on differentiation in experimental teratomas in vivo . To this end, Sox17-DsRed-Ctrl-KD, Sox17-DsRed-Klf4-KD and Sox17-DsRed-Klf5-KD ES cells were injected into the testes of severe combined immunodeficient (SCID) mice. After 3 weeks, expression of endoderm and mesoderm markers was analysed by quantitative real-time PCR ( Fig. 7a ). Compared with the control, teratomas generated with Klf4-KD ES cells displayed elevated expression of the early endodermal markers Sox7 , Sox17 , Dab2 , Gata4 , Fxyd3 , Foxa2 and HNF4α . In contrast, the teratomas generated with Klf5-KD ES cells displayed elevated expression of the mesodermal markers T , Mixl1 , Msx2 , Flk1 , Bmp2 , MyoD , Myf6, Tbx20 and Vegfr1 . In accord with the in vitro data, no difference was observed between Klf4-KD, Klf5-KD and control ES cells in the expression of ectodermal markers. 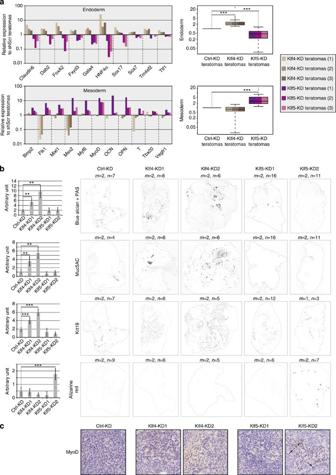Figure 7: Endodermal and mesodermal differentiation in experimental teratomas after Klf4 and Klf5 knockdown. (a) Quantitative real-time PCR analysis of mesodermal and endodermal lineage markers. Left panel: histogram showing the mRNA level of the indicated genes in Klf4-KD- and Klf5-KD-derived teratomas, after normalization to teratomas made with control-KD cells (shScr). Right panel: box plot histogram showing the average variations of the mRNA level of endodermal, ectodermal and mesodermal markers between control, Klf4-KD- and Klf5-KD-derived teratomas. ***P<0.001 using Kruskal–Wallis one-way ANOVA. (b) Teratomas sections immunolabelled with antibodies against gastric Mucin5AC, cytokeratin 19 (Krt19) or stained with alcian blue coupled with PAS to identify mucin-expressing epithelium, and alizarine red to identify osteogenic tissue. Right panels: digitalized sections of control, Klf4-KD1-, Klf4-KD2-, Klf5-KD1 and Klf5-KD2-derived teratomas, in which signal above background was converted to black dots and quantified with the ImageJ software. For each marker,nandmindicate the number of teratomas and number of sections analysed, respectively. Left panels: histogram representation of the mean staining intensity measured in n sections obtained from m teratomas. Error bars indicate standard deviation. *P<0.05; **P<0.01; ***P<0.001, using Student’st-test. (c) High magnification microphotographs showing positive cells in teratomas sections immunolabelled with antibody MyoD. Figure 7: Endodermal and mesodermal differentiation in experimental teratomas after Klf4 and Klf5 knockdown. ( a ) Quantitative real-time PCR analysis of mesodermal and endodermal lineage markers. Left panel: histogram showing the mRNA level of the indicated genes in Klf4-KD- and Klf5-KD-derived teratomas, after normalization to teratomas made with control-KD cells (shScr). Right panel: box plot histogram showing the average variations of the mRNA level of endodermal, ectodermal and mesodermal markers between control, Klf4-KD- and Klf5-KD-derived teratomas. *** P <0.001 using Kruskal–Wallis one-way ANOVA. ( b ) Teratomas sections immunolabelled with antibodies against gastric Mucin5AC, cytokeratin 19 (Krt19) or stained with alcian blue coupled with PAS to identify mucin-expressing epithelium, and alizarine red to identify osteogenic tissue. Right panels: digitalized sections of control, Klf4-KD1-, Klf4-KD2-, Klf5-KD1 and Klf5-KD2-derived teratomas, in which signal above background was converted to black dots and quantified with the ImageJ software. For each marker, n and m indicate the number of teratomas and number of sections analysed, respectively. Left panels: histogram representation of the mean staining intensity measured in n sections obtained from m teratomas. Error bars indicate standard deviation. * P <0.05; ** P <0.01; *** P <0.001, using Student’s t -test. ( c ) High magnification microphotographs showing positive cells in teratomas sections immunolabelled with antibody MyoD. Full size image To investigate whether knockdown of Klf4 and Klf5 increases the yield of mesodermal and endodermal structures, respectively, teratoma sections were stained with alcian blue coupled to periodic acid Schiff to identify mucin-expressing epithelium, and alizarin red to identify osteogenic tissue. Teratoma sections were also immunolabelled with antibodies against gastric Mucin5AC, cytokeratin 19 (Krt19), Clara cell protein 10 (CC10), surfactant protein C (SP-C), MyoD and smooth muscle actin, and subsequently digitalized for signal quantification ( Fig. 7b,c , Supplementary Fig. 8 ). Compared with the control, teratomas generated with Klf4-KD ES cells contained larger regions expressing the endoderm markers (mucins, Muc5AC and Krt19). Both markers were observed within the gland structures typical of endoderm differentiation. In contrast, no difference was observed between the control and Klf5-KD cells-derived teratomas for these markers. In a mirror image, teratomas generated with Klf5-KD cells exhibited considerably more of the mesoderm-derived tissues, namely alizarin red-positive bone tissue (only observed in the Klf5-KD2 cells-derived teratomas), and MyoD-positive nuclei. In the Klf5-KD cells-derived teratomas, the MyoD-positive cells clustered in muscle-like structures that could not be observed in control and Klf4-KD cells-derived teratomas. Of note, the lung markers CC10 and SP-C, and the smooth muscle marker smooth muscle actin, showed no difference between the five groups of teratomas. This latter observation indicates that not all endoderm and mesoderm lineages are biased by Klf knockdown in the teratomas analysed. Together these results show that Klf4 and Klf5 knockdown impairs lineage choice in the experimental teratomas in vivo . In accord with the in vitro data, Klf4 knockdown upregulates markers of early endodermal differentiation and coaxes differentiation into glandular tissues. In a mirror image, Klf5 knockdown upregulates markers of early mesodermal differentiation, and coaxes differentiation into bone and skeletal muscle tissues. In this study, we have shown that Klf4 and Klf5 exert distinct roles in the inhibition of mesoderm and endoderm differentiation in mouse ES cells. Our results indicate that Klf4 inhibits differentiation towards visceral and definitive endoderm, whereas Klf5 inhibits differentiation towards mesoderm. Thus, the additive functions of Klf4 and Klf5 secure ES cell propagation by inhibiting endoderm and mesoderm differentiation ( Fig. 8 ). 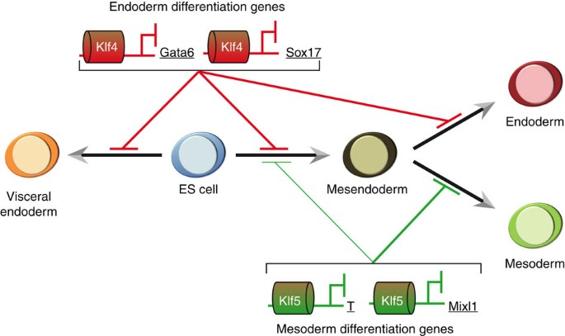Figure 8: Additive function of Klf4 and Klf5 secures ESC propagation by inhibiting endoderm and mesoderm differentiation.  Figure 8: Additive function of Klf4 and Klf5 secures ESC propagation by inhibiting endoderm and mesoderm differentiation. Full size image Inhibition of endodermal differentiation by Klf4 is likely to result from the repression of endoderm-specific regulators, including Gata4 , Gata6 , Sox7 , Sox17 , Foxa2 , Amnionless and Dab2 . Overexpression of Gata4 and Gata6 is known to induce differentiation of mouse ES cells to PE [40] , [41] . Forced expression of Sox17 in human ES cells produces definitive endoderm progenitors [30] , whereas overexpression in mouse ES cells directly activates genes functioning in differentiation towards both an extraembryonic and a definitive cell fate [29] , [31] . Forced expression of Sox7 has been shown to induce differentiation of F9 embryonal carcinoma cells to parietal endoderm [26] . The role of Amn and Dab2 in ES cell differentiation has not been investigated, but their role during early embryo development is relatively well characterized. Amn is expressed in the visceral endoderm and regulates the BMP signalling pathway that controls the production of trunk mesoderm [42] . Dab2 is first expressed in the PE of the 4.5-day blastocyst. Disruption of Dab2 results in disorganization of the visceral endoderm and subsequent developmental arrest at 6.5 days of gestation [43] . Thus, all of these genes are involved in the formation and/or organization of endodermal structures. They were activated up to 7.5-fold upon only a 2-fold reduction in Klf4 RNA level in self-renewing ES cells, suggesting that Klf4 is a key regulator of those endodermal markers. Promoter study has shown that all of these genes have binding sites for Klf4 in their promoter sequence. Moreover, Klf4 inhibits the expression of Gata6 expression in a transient expression assay. Thus, we conclude that inhibition of Gata6 is one mechanism by which Klf4 inhibits differentiation of ES cells to endoderm. Of note, ChIP-Seq and ChIP–PCR experiments have revealed the ability of Klf4 to bind equally the promoters of Gata6 , Sox17 , Mixl1 and T. However, only the Gata6 and Sox17 were upregulated by Klf4 knockdown, and downregulated by Klf4 overexpression ( Fig. 1 ). Moreover, only Klf4 repressed the Gata6 promoter in the transient expression assay ( Fig. 6c ). This finding suggests that the specificity of Klf action is dictated by competitive binding of Klf4 and Klf5 to their cognate binding site and by Klf-specific co-factors required for transcriptional activation. In a mirror image, our results indicate that the inhibition of mesodermal differentiation by Klf5 is likely to result at least partially from the repression of the mesoderm-specific regulator Mixl1 . It was shown that the ectopic induction of Mixl1 in ES cells results in premature activation of Gsc , and increased the frequency of Flk1 + c-kit + hematopoietic progenitors observed in day 4 EBs [44] . Our observation that the ES-Gsc gfp Sox17 huCD25 -Klf5-KD clones increased Gsc expression in comparison with control cells ( Fig. 4c,d ) is consistent with a regulation of Gsc by Mixl1 . Mixl1 was upregulated 2.5-fold upon a twofold reduction in Klf5 RNA level in self-renewing ES cells. Our promoter study showed that Mixl1 has binding sites for Klf4 and Klf5 in its promoter sequence, and the binding of Klf5 is much stronger than the binding of Klf4. Moreover, Klf5 inhibits expression of Mixl1 in a transient expression assay. Thus, we conclude that inhibition of Mixl1 is one mechanism by which Klf5 inhibits differentiation of ES cells to mesoderm. The finding that Klf5 preferentially inhibits mesodermal differentiation in ESCs is at odds with a previous study showing that loss of Klf5 resulted in increased Sox17 expression in the PE in Klf5 −/− 3.5 dpc blastocysts and the Klf5 −/− cells preferentially contributed to the Sox17 + PE lineage in Klf5 +/+ / Klf5 −/− chimeric embryos [45] . The same study also showed that outgrowths from the Klf5 −/− ICM failed to form an ICM/pluripotent colony, had very few Oct4 + cells, but showed an increase in the percentage of Sox17 + PE cells. The discrepancy between our study and the study of Lin et al. [45] may be explained by the capacity of other Klf members to rescue the loss of Klf5 function in ES cells. In the pre-implantation embryo, the loss of Klf5 results in developmental arrest prior to the expanded blastocyst stage caused by defective trophectoderm development and reduced expression of Oct4 and Nanog [14] , [45] . In contrast, Klf2 , Klf4 and Klf5 are known to have redundant functions in the maintenance of the undifferentiated state of ES cells, as shown by the capacity of each one of them, when overexpressed, to rescue pluripotency after Klf2 / Klf4 / Klf5 triple knockdown-induced differentiation [17] . We speculate that rescue of the Klf5 function by Klf2 and Klf4 allows the self-renewing ES cells to overcome PE differentiation, revealing an as yet unknown function of Klf5 in the inhibition of mesodermal differentiation. At first sight, it is intriguing that Klf4 inhibits definitive endoderm differentiation, and Klf5 mesodermal differentiation, given that the sharp drop in Klf4 and Klf5 expression occurs as early as days 1–2 of EB differentiation [10] , whereas both the drop in Nanog , Oct4 and Sox2 expression and the rise in definitive endoderm and mesoderm markers takes place no earlier than days 3–4 ( Fig. 3c , and Supplementary Fig. 5 ). One possible explanation could be the co-repression of endoderm and mesoderm-specific promoters by Nanog, Oct4 and Sox2 pluripotency factors. The drop in Klf4 and Klf5 expression would prime ES cells for commitment into endoderm and mesoderm, respectively, but this commitment would become effective only after Nanog, Oct4 and Sox2 have been fully extinguished. shRNA design and plasmid construction Interfering lentiviral vectors expressing shRNAs specific to the coding sequences of Klf4 and Klf5 have previously been described [10] . shRNA sequences specific to the 3′untranslated region of Klf4 and Klf5 mRNAs were designed using the si DESIGN Center application of Dharmacon ( http://www.dharmacon.com ) ( Supplementary Table 1 ). For each targeted gene, five independent shRNA 3′UTR were cloned into pENTRY (Invitrogen, Ref. K4943-00), and the resulting pENTRY-shRNA vectors transfected into CGR8 ES cells so as to measure the interference by real-time PCR. For each targeted gene, the shRNA sequence, which showed the highest interference in the transient transfection assay, were subcloned into pLenti6/BLOCK-iT-PGKneo r [10] . To generate lentivectors expressing Klf4 and Klf5, mouse Klf4 and Klf5 cDNA were amplified from a mouse ESC cDNA library, using primers containing BamHI and HindIII sites. The resulting fragments containing the Klf4 and Klf5 coding sequences were subcloned between the BamHI and HindIII sites in pGAE-CAG-eGFP-WPRE [46] to generate pGAE-Klf4 and pGAE-Klf5. For the construction of pGL4-Gata6Pro , the fragment containing the −4,528 to +1,844 region of the Gata6 gene was digested from the pBS-LacZ-Gata6 [47] with SacI(Blunt) and BglII and subcloned between the HindIII(blunt) and BglII sites of pGL4.10 Luc2 (Promega). For construction of pGL4-Mixl1Pro , the −858 to +1 region of the Mixl1 gene was synthesized (Geneart) and subcloned between the KpnI and XhoI sites of pGL4.10 Luc2 . ES cell culture and differentiation All ES cell lines were routinely cultured in Glasgow’s modified Eagle’s medium (GMEM) supplemented with 10% fetal calf serum (PerbioScience CRC0406) and 1,000 U ml −1 of LIF. To induce differentiation, cells were allowed to form aggregates in hanging drops in ES cell medium without LIF (100 cells per drop). After 2 days, EBs were collected and further grown in suspension for 1–10 days in non-adherent Petri dishes. Differentiation into visceral endoderm was induced by culturing the cells on gelatin-coated dishes in SF03 serum-free culture medium at high-cell density (10 4 cells per cm 2 ). Differentiation into mesendoderm/definitive endoderm was induced by culturing cells on collagen IV-coated dishes in SF03 supplemented with 10 ng ml −1 human activin A at low-cell density (10 3 cells per cm −2 ) [27] . Differentiation was performed in α Modified Eagle’s Medium to enhance mesoderm differentiation [39] . Generation of lentiviral vectors and infection of target cells For Klf4 and Klf5 knockdown, lentiviral vectors were produced using the BLOCK-iT lentiviral RNA interference expression system (Invitrogen, Ref. K4944-00) according to the manufacturer’s instructions. To produce SIV-derived lentivectors, 293T cells were transfected with a mixture of DNA containing 7.5 μg of a pGRev plasmid encoding for the vesicular stomatitis virus glycoprotein envelope; 4 μg of a pSIV3 + plasmid encoding for the gag, pol, tat and rev proteins; and 11.5 μg of vector plasmids ( pGAE-CAG-Klf4-WPRE and pGAE-CAG-Klf5-WPRE ) using the calcium phosphate precipitation technique. For infection, CGR8 were plated at a density of 10 4 cells in 24-well plates in 1 ml of medium composed of 100 μl of ES cell medium and 900 μl of culture supernatant from virus-producer cells. After 48 h, ES cells were trypsinized, re-plated at 10 4 cells per gelatin-coated 10 mm tissue culture dish and further cultured for 6 days in complete ES cell medium supplemented with 250 μg ml −1 of G418 and 1,000 U ml −1 LIF [48] . Real-time PCR RNA was extracted using RNAeasy kits with on-column DNAse digestion and reverse transcription performed with MuMLV-RT (Promega), according to the manufacturer’s recommendations. Oligonucleotide sequences are given in Supplementary Table 2 . Quantitative PCR was performed using the LightCycler 1.5 system and the LightCycler Fast Start DNA Master SYBR Green I kit (Roche Applied Science) according to the manufacturer’s instructions. All normalizations were performed with β-actin . Generation of teratomas and immunolabelling ESCs were inoculated beneath the testicular capsule of 7-week-old SCID males (CB17/SCID; Charles River Laboratories), 5–10 weeks. Later, mice were euthanized, and lesions were surgically removed. All animal studies were conducted according to the guidelines and following approval by the Ministry of higher education and research (C2EA42-13-02-0402-07). Teratomas were fixed in formaldehyde, embedded in paraffin wax and sectioned. Immunostaining was performed with standard protocol. Antigen retrieval was performed by stem heater boiling in citrate buffer pH 6. Incubation with the primary antibodies was performed overnight at 4 °C. The primary antibodies used are the following: MyoD1, mouse monoclonal, Abcam ab1614 (40 μg ml −1 ); Krt19, rat monoclonal, Developmental Studies Hybridoma Bank #TROMA-III, 1DB-001-0000868971 (10 μg ml −1 ); SP-C, rabbit polyclonal, Millipore AB3786 (1 μg ml −1 ); CC10, goat polyclonal, Santa Cruz Biotechnology sc-9772 (0.2 μg ml −1 ); Muc5AC (45M1) (0.2 μg ml −1 ) [49] . horseradish peroxidase-conjugated secondary antibodies (DAKO) were used, and 3,3'-diaminobenzidine (DAB, DAKO) was used as a chromogen for visualization of positive cells. Nuclei were counterstained with hematoxylin. Alcian blue coupled to periodic acid Schiff (PAS) staining was used to label mucins, and alizarin red (AR) staining was used to mark the osteogenic lineage [50] . To quantify labelling, teratoma sections were digitalized using the Pannoramic Viewer software (3DHistech). Colour images with DAB (brown), Alcian blue/PAS (dark blue+pink) and AR (pink) staining were subsequently converted to grey scale images using Photoshop. The grey intensity was quantified with ImageJ in each section, and subsequently normalized to the section area. Note that testicular and necrotic tissues were excluded from the quantification. Flow cytometry For analysis by flow cytometry, EBs were dissociated with cell dissociation buffer (GIBCO-BRL). Cells were stained using various combinations of antibodies. Antibodies used in this study were previously described [27] , [38] : APC-anti-human CD25 mAb (M-A251, Becton-Dickinson & Co; 5 μl 10 −6 cells), fluorescein-anti-mouse E-Cadherin mAb (FAB7481F, R&D systems; 2.5 μg ml −1 ), APC-anti-mouse CD140a (PDGFRα) mAb (17–1401, eBioscience; 5 μg ml −1 ) and APC-anti-mouse Flk1 mAb (560070, BD pharmingen; 5 μg ml −1 ). Cells were analysed with a FACS Canto II (Becton-Dickinson). Data were recorded and analysed with DiVa software. Microarrays and bioinformatics Total RNAs from ES cells was prepared with the Qiagen column kit (Qiagen) and treated with DNAse (5 U per 100 mg RNA, Qiagen). Biotinylated cRNA was prepared according to the standard Affymetrix protocol (Expression Analysis Technical Manual, 1999; Affymetrix). In brief, double-stranded cDNA was synthesized from 10 μg total RNA using the SuperScript Choice System from Invitrogen and the Affymetrix T7-(dT) 24 primer that contains a T7 RNA polymerase promoter attached to a poly-dT sequence. The cDNA was transcribed into biotin-labeled cRNA using the IVT Megascript T7 kit (Ambion), Biotin 11-CTP and Biotin 16-UTP (PerkinElmer). cRNA purification, fragmentation and hybridization on the Mouse Genome 430 2.0 Array was done according to Affymetrix recommendations. The image data were analysed with the GeneChip Operating Software using Affymetrix default analysis settings. Arrays, after passing the quality control, were commonly RMA normalized [51] . Expression differences between conditions were evaluated using ANOVA, t -test statistic and Benjamini-Hochberg false-discovery rate correction. K-mean clustering and hierarchical average linkage clustering was performed using Cluster version 2.11 (ref. 53 ). ChIP ChIPs for Klf4- and Klf5-expressing cells were performed using previously described protocols [53] . In brief, cells were cross-linked with 1% formaldehyde for 10 min at room temperature and formaldehyde was inactivated by the addition of 125 mM glycine. Chromatin from mouse ES cells expressing Klf4 and Klf5 was sonicated to a length of ~250–500 bp, and subsequently immunoprecipitated using custom-made Klf4 or Klf5 antibodies generously provided by Dr Huck-Hui Ng [17] , [21] . Samples were sequenced using the Illumina Genome Analyzer IIx platform. Quantitative PCR analyses were then performed for each ChIP experiment in real time using the ABI PRISM 7900 sequence detection system and SYBR Green master mix. ChIP–PCR data are presented in percent of input with the immunoglobulin G control. Relative occupancy values were calculated by determining the apparent immunoprecipitation efficiency (ratio of the amount of immunoprecipitated DNA to that of the input sample) and normalized to the level observed at a control region, which was defined as 1.0. Primer sequences are listed in Supplementary Table 2 . ChIP-Seq reads were aligned using the Eland software to NCBI build 37 (mm9) of the mouse genome. The MACS programme (version 1.4) [54] was used to detect peaks of ChIP enrichment and run with the default settings using a tag size of 35 and a band width of 280. Redundant reads that could result from the overamplification of ChIP-DNA were removed, and peak enrichment was calculated relative to the genome background. A threshold of P =10 −10 was used to call significant peaks. An input control sample was also included to eliminate nonrandom enrichment. ChIP-seq was performed on one replicate. The findMotifsGenome.pl programme from software suite HOMER was used to find de novo motifs using windowBed ( http://code.google.com/p/bedtools/ ). Primers for PCR are as follows: Sox17-F:5′-ATTAACTTCGGGGGCTCATT-3′; Sox17-R:5′-CGGGAGCAGTTTACTTCCTG-3′; T-F:5′-CTTTGATGGAGGTGCAAACA-3′; T-R:5′-CCCCTCCCCATAAATACAGC-3′; Mixl1-F:5′-GAATAATCGCTTCCGCTGAC-3′, Mixl1-R:5′-AGAGGGGGTTCTGTCCAAGT-3′; Gata6-F:5′-AGTTTTCCGGCAGAGCAGTA-3′, Gata6-R:5′-AGGAGGAAACAACCGAACCT-3′. Reporter assay For plasmid transfection, 400 ng of pGL4.10 Luc2 reporter plasmid were mixed with 0.6 μl of lipofectamine (Life Technologies) in 25 μl of Opti-MEM. The resulting mixture was added to CGR8 ES cells at a density of 2.5 × 10 4 cells per 96 wells in 1.5 ml of medium. The pRL-TK plasmid (Promega), which expresses Renilla , was co-transfected as an internal control (1 ng per well) with other plasmids. At 48 h post transfection, luciferase assays were performed using the dual-luciferase assay system (Promega). Activities of both firefly and Renilla luciferases were measured using a Glomax microplate luminometer (Promega). Relative luciferase was calculated by normalizing firefly luciferase activity (reporter) to Renilla luciferase activity (internal control). Accession codes: Microarray data are available in the arrayexpress database ( http://www.ebi.ac.uk/arrayexpress ) under the accession numbers E-MTAB-1838 and E-MTAB-1839. ChIP-seq data have been deposited at Gene Expression Omnibus under accession number GSE49848 . How to cite this article: Aksoy, I. et al. Klf4 and Klf5 differentially inhibit mesoderm and endoderm differentiation in embryonic stem cells. Nat. Commun. 5:3719 doi: 10.1038/ncomms4719 (2014).